The neural circuits and sensory channels mediating harsh touch sensation inCaenorhabditis elegans Most animals can distinguish two distinct types of touch stimuli: gentle (innocuous) and harsh (noxious/painful) touch, however, the underlying mechanisms are not well understood. Caenorhabditis elegans is a useful model for the study of gentle touch sensation. However, little is known about harsh touch sensation in this organism. Here we characterize harsh touch sensation in C. elegans . We show that C. elegans exhibits differential behavioural responses to harsh touch and gentle touch. Laser ablations identify distinct sets of sensory neurons and interneurons required for harsh touch sensation at different body segments. Optogenetic stimulation of the circuitry can drive behaviour. Patch-clamp recordings reveal that TRP family and amiloride-sensitive Na + channels mediate touch-evoked currents in different sensory neurons. Our work identifies the neural circuits and characterizes the sensory channels mediating harsh touch sensation in C. elegans , establishing it as a genetic model for studying this sensory modality. The sense of touch is a universal phenomenon found in nearly every organism [1] . In animals, specialized sensory systems have been evolved to detect and react to touch, which are essential for their survival and reproduction [2] . Most animals can distinguish at least two distinct types of touch stimuli: gentle touch and harsh touch, with the former being harmless and sometimes pleasant and the latter unpleasant and often painful [2] . In mammals, the myelinated Aβ sensory nerves detect gentle touch, whereas the lightly myelinated Aδ and non-myelinated C fibres sense harsh touch [2] . However, unlike photosensation and chemosensation that have been extensively characterized in mammals, little is known about the molecular mechanisms of touch sensation [1] . For example, the central players in touch sensation, the mechanosensitive channels that are believed to convert forces into electrical responses, have not been identified in mammals. The nematode Caenorhabditis elegans is a widely used model organism for sensory transduction such as touch sensation, chemosensation and photosensation [1] , [3] , [4] , [5] , [6] . In particular, C. elegans is renowned for its success in studying the mechanisms of gentle touch sensation [1] . A group of sensory neurons (ALM, AVM and PLM) sense gentle touch in the body of the worm, whereas ASH, OLQ and FLP detect gentle touch at the nose tip [1] , [7] . A saturated forward genetic screen has identified a mechanotransduction channel complex that senses gentle body touch, with the epithelial sodium channel (ENaC) family proteins MEC-4/MEC-10 forming the channel pore, and MEC-6 and MEC-2 linking the channel to the extracellular matrix and intracellular cytoskeleton, respectively [1] , [8] . Remarkably, many of the genes in this complex are evolutionarily conserved, which has prompted characterization of the function of their homologues in gentle touch sensation in mammals. Indeed, the mammalian homologue of MEC-2 and MEC-4 has recently been reported to have an important role in gentle touch sensation and pressure sensation in mice, respectively [9] , [10] . However, unlike gentle touch sensation, little is known about harsh touch sensation in C. elegans . The behavioural responses to harsh touch have not been clearly defined. Although one neuron (PVD) has been found to act in harsh touch sensation [11] , [12] , the majority of the circuitry is unknown. Here, we characterize harsh touch sensation in C. elegans by defining the behavioural responses to harsh touch and by dissecting the underlying neural circuits and genes. We show that as is the case with mammals, C. elegans exhibits differential behavioural responses to harsh and gentle touch and uses distinct sensory neurons to detect harsh and gentle touch. Optogenetic stimulation of the circuitry can mimic behavioural responses. Through electrophysiological recording, we show that both transient receptor potential (TRP) family and amiloride-sensitive Na + channels mediate mechanosensitive currents, but in different sensory neurons. Calcium imaging of the circuitry reveals a neuronal correlate for harsh and gentle touch sensation. Our results establish a framework for understanding the mechanisms of harsh touch sensation in a genetic model organism. Differential behavioural responses to harsh and gentle touch Eyelash is commonly used to deliver gentle touch to the anterior and posterior body of the animal with a force in the range of 1–10 μN, which triggers backward and forward movement, respectively [13] . To deliver harsh touch, we used a platinum wire pick with a force of 100–200 μN ( Fig. 1a ). Stronger forces (>500 μN) often caused physical damages to the animal, manifested by a sluggish or loss of response in the following trials. Animals reacted to anterior harsh touch by initiating backward movement and to posterior harsh touch by initiating forward movement ( Fig. 1b , Supplementary Fig. S1a and Movies 1 , 2 ); however, the responses were much more robust than gentle touch responses. As a direct comparison, we focused on the anterior touch response as it is relatively straightforward to quantify this response by measuring the distance (number of head swings) of backward movement. Under our conditions, gentle touch-triggered backward movement lasted an average of 1.7±0.2 head swings, which was usually followed by forward movement without a direction change ( Fig. 1c,d ). By contrast, harsh touch-evoked backward movement lasted an average of 5.1±0.4 head swings, which was often followed by a direction change ( Fig. 1c,d ). Such direction change ensures that the animal would not return to its previous location. This avoidance response may help animals to effectively avoid hazardous environments. Thus, C. elegans shows differential behavioural responses to gentle and harsh touch. 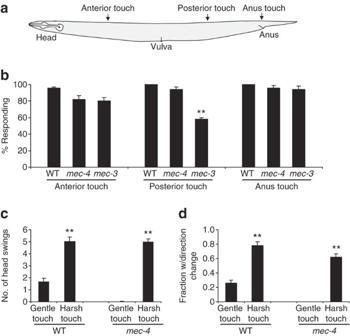Figure 1: Animals exhibit differential behavioural responses to harsh touch and gentle touch. (a) A schematic illustrating the location of harsh touch stimuli delivered to different body segments. (b) Response of WT,mec-4(e1611)andmec-3(e1338)worms to anterior, posterior and anus harsh touch.mec-4(e1611)andmec-3(e1338)worms were outcrossed six and four times, respectively. The non-outcrossed CGC strain CB1338 ofmec-3(e1338)was a bit unhealthy and showed reduced responses (Supplementary Fig. S1).n=10. **P<0.0001 (ANOVA with Bonferroni test). Error bars: s.e.m. (c) Animals respond to harsh touch more robustly than gentle touch. The number of head swings of backward movement triggered by anterior gentle and harsh touch was scored. **P<0.0001 (t-test; harsh touch versus gentle touch). However, harsh touch data frommec-4(e1611)mutant and wild-type under were not significantly different.n=10. Error bars: s.e.m. (d) The frequency of direction change following backward movement triggered by anterior harsh touch and gentle touch. A direction change was defined as a ≥90° turn from the previous locomotion direction. **P<0.0001 (t-test; harsh touch versus gentle touch). However, harsh touch data frommec-4(e1611)mutant strain and wild-type were not significantly different.n=10. Error bars: s.e.m. WT, wild type. Figure 1: Animals exhibit differential behavioural responses to harsh touch and gentle touch. ( a ) A schematic illustrating the location of harsh touch stimuli delivered to different body segments. ( b ) Response of WT, mec-4(e1611) and mec-3(e1338) worms to anterior, posterior and anus harsh touch. mec-4(e1611) and mec-3(e1338) worms were outcrossed six and four times, respectively. The non-outcrossed CGC strain CB1338 of mec-3(e1338) was a bit unhealthy and showed reduced responses ( Supplementary Fig. S1 ). n =10. ** P <0.0001 (ANOVA with Bonferroni test). Error bars: s.e.m. ( c ) Animals respond to harsh touch more robustly than gentle touch. The number of head swings of backward movement triggered by anterior gentle and harsh touch was scored. ** P <0.0001 ( t -test; harsh touch versus gentle touch). However, harsh touch data from mec-4(e1611) mutant and wild-type under were not significantly different. n =10. Error bars: s.e.m. ( d ) The frequency of direction change following backward movement triggered by anterior harsh touch and gentle touch. A direction change was defined as a ≥90° turn from the previous locomotion direction. ** P <0.0001 ( t -test; harsh touch versus gentle touch). However, harsh touch data from mec-4(e1611) mutant strain and wild-type were not significantly different. n =10. Error bars: s.e.m. WT, wild type. Full size image We also tested the anus area, as C. elegans recruits a different set of neurons for harsh touch sensation in this area (see below). Animals reacted to anus touch by initiating forward movement ( Fig. 1b ). Finally, we tested the middle segment (vulva touch). Unlike other body segments, animals reacted to vulva touch by initiating either forward or backward movement with a bias towards forward movement ( Supplementary Fig. S1b ). Because of this, we focused our efforts on characterizing anterior, posterior and anus touch responses. Gentle touch mutants retain harsh touch responses We tested the gentle touch-insensitive mutant mec-4(e1611) in which all gentle-touch sensory neurons degenerate [14] . As reported [11] , although insensitive to gentle touch , this mutant was sensitive to harsh touch ( Fig. 1b ; Supplementary Movies 3 , 4 ). Specifically, the number of head swings of backward movement triggered by anterior harsh touch and the frequency of direction change following backward movement were similar to those observed in wild-type, suggesting that animals lacking gentle touch sensitivity retain normal harsh touch responses ( Fig. 1b–d ). Thus, C. elegans may depend on different neurons for harsh touch sensation. Interneurons required for harsh touch responses To identify the neural circuits underlying harsh touch sensation, we applied a laser ablation approach. We first examined the interneurons. The interneuron circuits underlying gentle touch behaviour have been well characterized [15] . The backward command interneurons AVA and AVD together are required for anterior gentle touch response, whereas the forward command interneuron PVC mediates posterior gentle touch response [15] . The other backward command interneuron AVE, however, is dispensable for gentle touch behaviour [15] ( Fig. 2a ). The backward and forward command interneurons drive backward and forward movement by controlling downstream ventral cord motor neurons, respectively [15] . We killed these interneurons individually and in combination with a laser microbeam. Although ablation of AVA, AVD and AVE individually only led to a modest defect in anterior harsh touch response, animals lacking AVA, AVD and AVE in combination failed to move backwards upon anterior harsh touch ( Fig. 2b ); yet these animals maintained normal posterior and anus harsh touch responses ( Supplementary Fig. S2a,b ). Thus, AVA, AVD and AVE are specifically required for anterior harsh touch response. 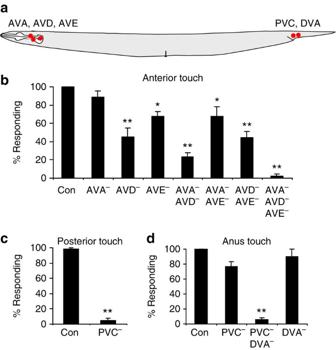Figure 2: Identification of the interneurons required for harsh touch behaviour. (a) A schematic illustrating the position of interneuron cell bodies. (b) AVA, AVD and AVE are required for mediating anterior but not posterior or anus harsh touch response. *p<0.02. **p<0.0001 (ANOVA with Bonferroni test compared with control).n≥5. Error bars: s.e.m. (c) PVC is required for mediating posterior but not anterior or anus harsh touch response. **P<0.0001 (t-test).n≥12. Error bars: s.e.m. (d) PVC and DVA together are required for mediating anus harsh touch response. **P<0.0001 (ANOVA with Bonferroni test compared with control).n≥4. Error bars: s.e.m. Figure 2: Identification of the interneurons required for harsh touch behaviour. ( a ) A schematic illustrating the position of interneuron cell bodies. ( b ) AVA, AVD and AVE are required for mediating anterior but not posterior or anus harsh touch response. *p<0.02. **p<0.0001 (ANOVA with Bonferroni test compared with control). n ≥5. Error bars: s.e.m. ( c ) PVC is required for mediating posterior but not anterior or anus harsh touch response. ** P <0.0001 ( t -test). n ≥12. Error bars: s.e.m. ( d ) PVC and DVA together are required for mediating anus harsh touch response. ** P <0.0001 (ANOVA with Bonferroni test compared with control). n ≥4. Error bars: s.e.m. Full size image Similarly, animals lacking the forward command interneuron PVC failed to move forward upon posterior harsh touch ( Fig. 2c ), but responded normally to anterior harsh touch ( Supplementary Fig. S2c,d ). Thus, PVC is required for posterior harsh touch response. However, PVC-ablated animals can still move forward upon anus touch, albeit at a reduced frequency ( Fig. 2d ). Apparently, additional interneurons must contribute to anus response. We considered those in the anus area that form synaptic connections with ventral cord motor neurons. DVA came to our attention, as it synapses onto the B type ventral cord motor neurons that drive forward locomotion [16] . Although ablation of DVA alone led to a slight reduction in anus response, animals with both PVC and DVA ablated were unable to move forward upon anus touch, indicating that DVA and PVC together are required for anus response ( Fig. 2d and Supplementary Fig. S2e,f ). Sensory neurons required for anterior harsh touch sensation We then sought to identify the sensory neurons required for harsh touch sensation. To eliminate gentle touch responses, we killed the anterior gentle touch neurons ALM/AVM and the posterior gentle touch neuron PLM on top of all of the ablations aimed at identifying anterior and posterior/anus harsh touch sensory neurons, respectively. To identify the sensory neurons required for detecting anterior harsh touch, we considered candidates that are located in the anterior body and also form synaptic connections with the anterior interneurons AVA/AVD/AVE ( Fig. 3a ). BDU and SDQR fall into this category [16] . Laser ablation of BDU or SDQR led to a significant reduction in anterior harsh touch response ( Fig. 3b ). Killing BDU together with SDQR, but not with SDQL, yielded a more severe defect ( Fig. 3b and Supplementary Fig. S3 ). Nevertheless, these animals retained an ∼ 20% response rate ( Fig. 3b ). These results indicate that although BDU and SDQR have an important role in anterior harsh touch sensation, other sensory neurons are also involved. 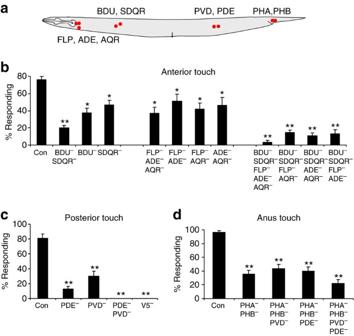Figure 3: Identification of the sensory neurons required for harsh touch behaviour. (a) A schematic illustrating the location of sensory neuron cell bodies. (b) Two groups of sensory neurons are required for mediating anterior harsh touch response. The anterior gentle touch sensory neurons ALM and AVM were killed in all ablations. *P<0.03. **P<0.0001 (ANOVA with Bonferroni test compared with control).n≥9. Error bars: s.e.m. (c) PVD and PDE together are required for mediating posterior harsh touch response. The posterior gentle touch sensory neuron PLM was killed in all ablations. V5 is the precursor cell of PVD and PDE. **P<0.0001 (ANOVA with Bonferroni test compared with control).n≥7. Error bars: s.e.m. (d) PHA/PHB is important for mediating anus harsh touch response. PLM was killed in all ablations. **P<0.0001 (ANOVA with Bonferroni test compared with control).n≥9. Error bars: s.e.m. Figure 3: Identification of the sensory neurons required for harsh touch behaviour. ( a ) A schematic illustrating the location of sensory neuron cell bodies. ( b ) Two groups of sensory neurons are required for mediating anterior harsh touch response. The anterior gentle touch sensory neurons ALM and AVM were killed in all ablations. * P <0.03. ** P <0.0001 (ANOVA with Bonferroni test compared with control). n ≥9. Error bars: s.e.m. ( c ) PVD and PDE together are required for mediating posterior harsh touch response. The posterior gentle touch sensory neuron PLM was killed in all ablations. V5 is the precursor cell of PVD and PDE. ** P <0.0001 (ANOVA with Bonferroni test compared with control). n ≥7. Error bars: s.e.m. ( d ) PHA/PHB is important for mediating anus harsh touch response. PLM was killed in all ablations. ** P <0.0001 (ANOVA with Bonferroni test compared with control). n ≥9. Error bars: s.e.m. Full size image To identify the sensory neurons that function redundantly with BDU and SDQR in the anterior circuit, we considered FLP, AQR and ADE that form synaptic connections with AVA/AVD/AVE and are located close to the terminal end of the pharynx [16] . Unlike BDU and SDQR, these three sensory neurons are ciliated neurons [16] . Although the sensory cilium of FLP is located at the nose tip, this neuron has multiple dendritic branches extending into the anterior body [16] , [17] . This appears to be a distinct feature pertaining to these three sensory neurons, as other head sensory neurons send their sensory endings to the nose tip [16] . Laser ablation of FLP, AQR and ADE together resulted in a significant reduction in anterior response, but did not abolish it ( Fig. 3b ). Thus, these three ciliated sensory neurons are important, although not required, for anterior harsh touch sensation. We therefore ablated these two distinct groups of neurons together. Laser ablation of BDU, SDQR, FLP, ADE and AQR together virtually eliminated anterior response ( Fig. 3b ). As a control, the ablated animals (also lacking gentle touch neurons) responded normally to posterior and anus harsh touch ( Supplementary Fig. S4 and S5 ). Thus, these sensory neurons together are specifically required for anterior harsh touch sensation. Sensory neurons required for posterior harsh touch sensation To identify the sensory neurons required for posterior harsh touch sensation, we examined those that are located in the posterior body and form synaptic connections with the posterior interneuron PVC. PVD and PDE fall into this category [16] ( Fig. 3a ). PVD is a non-ciliated multidendritic neuron regulating harsh touch sensation [12] , [17] , [18] , while PDE bears a sensory cilium [16] . PVD ablation led to a reduction in posterior response, but again it did not abolish it, indicating that additional sensory neurons are involved ( Fig. 3c ). Notably, ablation of PVD (together with gentle touch neurons) did not yield a defect in anterior response ( Supplementary Figs S3a, S4a and S6a ); nor did it affect anus response ( Supplementary Figs S4c and S6b ), indicating that PVD has a specific role in posterior harsh touch sensation. We also checked mec-3 mutant animals in which PVD is not fully differentiated [11] . Similarly, although mec-3 mutant animals showed a severe defect in sensing vulva touch, as previously reported [11] ( Supplementary Fig. S1b ), and exhibited a reduced response to posterior touch, this mutant retained normal sensitivity to anterior and anus harsh touch ( Fig. 1b ; Supplementary Fig. S1a ). Thus, PVD is not required for anterior, posterior or anus harsh touch sensation. Laser ablation of PDE also led to a strong defect in posterior response ( Fig. 3c ), indicating that PDE has an important role in this area. The observation that the loss of PVD or PDE reduced rather than abolished posterior response prompted us to reason that these two neurons may have a redundant role in posterior harsh touch sensation. Indeed, animals lacking both PVD and PDE failed to move forward upon posterior harsh touch ( Fig. 3c ). As a control, we killed PVD together with the other two posterior neurons PVM and SDQL, and found that these animals retained posterior response at a level similar to that observed in animals lacking PVD only ( Supplementary Fig. S3b ). Finally, animals lacking PVD, PDE and all gentle touch neurons, although defective in sensing posterior touch, responded normally to anterior and anus harsh touch ( Supplementary Fig. S4 ). Thus, PVD and PDE together are specifically required for posterior harsh touch response. Notably, instead of moving forward, animals lacking both PVD and PDE briefly “jerked” backwards upon posterior harsh touch ( Supplementary Movie 5 ). A similar phenomenon was observed in animals lacking the forward interneuron PVC. This suggests the presence of a competing circuit. As the behavioural output of this putative competing circuit was quite modest and only manifested in the absence of PVD and PDE, we did not explore it further in this study. Sensory neurons required for anus harsh touch sensation To identify the sensory neurons required for harsh touch sensation in the anus area, we first ablated the T cell, a precursor to a number of neurons in the anus area [19] , but did not detect a severe defect ( Supplementary Fig. S3c ). We then examined the ciliated sensory neurons in this area: PQR and PHA/PHB. Although loss of PQR did not lead to a notable defect ( Supplementary Fig. S3c ), ablation of PHA/PHB resulted in a significant reduction in anus response ( Fig. 3d ). As a control, no defect was detected in anterior or posterior responses in ablated animals ( Supplementary Fig. S4 and S7 ), indicating that PHA/PHB has a specific role in anus touch sensation. The observation that PHA/PHB-ablated animals retained residual ( ∼ 35%) anus response suggests the presence of additional sensory neurons in anus touch sensation. We considered several candidates. First, laser ablation of PHA/PHB and PQR together did not yield a more severe defect ( Supplementary Fig. S3c ), suggesting that PQR may not have an important role. This is consistent with the wiring pattern that PHA/PHB rather than PQR form synaptic connections with PVC and DVA [16] . Second, we tested DVA, which is unique in that it is both an interneuron and a sensory neuron (a proprioceptive neuron for body posture control) [20] , [21] . However, laser ablation of PHA/PHB and DVA together did not reveal a more severe defect in anus response ( Supplementary Fig. S3c ). Given that DVA and PVC are required for anus response ( Fig. 2d ), this result indicates that DVA may mainly function as an interneuron in the anus circuit. Finally, we considered the possibility that the posterior neurons PVD and PDE may have a role in anus touch sensation as the receptive field of these two neurons may extend to the anus area. PVD has sensory branches close to the anus [17] , [22] . Although PDE is physically distant from the anus, anus touch could slightly displace PDE cilium in distance. Indeed, laser ablation of PHA/PHB together with PVD and PDE further reduced the anus response rate to ∼ 20% ( Fig. 3d ). Although additional neurons are involved, these data identify PHA/PHB as the primary sensory neurons in mediating anus harsh touch sensation. Optogenetic stimulation of the circuitry can drive behaviour We tested whether stimulation of the identified sensory neurons can mimic harsh touch behavioural responses. We took an optogenetic approach by expressing ChR2, a light-gated non-selective cation channel [23] , [24] , in sensory neurons. ChR2 stimulation of the anterior neuron FLP initiated backward movement ( Fig. 4a ). Stimulation of the anterior neurons AQR, BDU and SDQR by ChR2 also triggered backward movement ( Fig. 4b ). 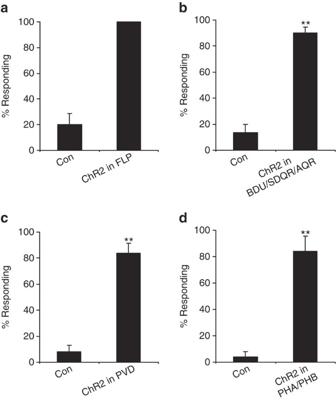Figure 4: Optogenetic stimulation of sensory neurons by ChR2 can drive behavioural responses. (a) ChR2 stimulation of FLP can drive backward movement. ChR2 was expressed in FLP as a transgene under themec-3promoter in thelite-1(xu7)mec-4(e1611)background. Themec-3promoter labels FLP, PVD and gentle touch neurons.lite-1(xu7)abolishes intrinsic phototaxis response5.mec-4(e1611)eliminates all gentle touch neurons14. We thus analysed FLP-positive animals in which PVD was killed by laser. Control animals were transgene-free siblings. **P<0.0001 (t-test).n≥5. Error bars: s.e.m. (b) ChR2 stimulation of BDU, SDQR and AQR can drive backward movement. ChR2 was expressed as a transgene under thegcy-35promoter in thelite-1(xu7)background. This promoter also labels URX and AVM in the head and anterior body45, so we analysed animals with URX and AVM ablated. Control animals were transgene-free siblings. **P<0.0001 (t-test).n≥6. Error bars: s.e.m. (c) ChR2 stimulation of PVD can drive forward movement. ChR2 was expressed in PVD as a transgene under themec-3promoter in thelite-1(xu7)mec-4(e1611)background. We analysed PVD-positive animals with FLP killed by laser. Control animals were transgene-free siblings. **P<0.0001 (t-test).n≥5. Error bars: s.e.m. (d) ChR2 stimulation of PHA/PHB can drive forward movement. ChR2 was expressed as a transgene under theocr-2promoter in thelite-1(xu7)background31. To avoid turning on the head neurons labelled by theocr-2promoter, we directed light pulses to the animal tail. Control animals were transgene-free siblings. **P<0.0001 (t-test).n≥5. Error bars: s.e.m. Figure 4: Optogenetic stimulation of sensory neurons by ChR2 can drive behavioural responses. ( a ) ChR2 stimulation of FLP can drive backward movement. ChR2 was expressed in FLP as a transgene under the mec-3 promoter in the lite-1(xu7)mec-4(e1611) background. The mec-3 promoter labels FLP, PVD and gentle touch neurons. lite-1(xu7) abolishes intrinsic phototaxis response [5] . mec-4(e1611) eliminates all gentle touch neurons [14] . We thus analysed FLP-positive animals in which PVD was killed by laser. Control animals were transgene-free siblings. ** P <0.0001 ( t -test). n ≥5. Error bars: s.e.m. ( b ) ChR2 stimulation of BDU, SDQR and AQR can drive backward movement. ChR2 was expressed as a transgene under the gcy-35 promoter in the lite-1(xu7) background. This promoter also labels URX and AVM in the head and anterior body [45] , so we analysed animals with URX and AVM ablated. Control animals were transgene-free siblings. ** P <0.0001 ( t -test). n ≥6. Error bars: s.e.m. ( c ) ChR2 stimulation of PVD can drive forward movement. ChR2 was expressed in PVD as a transgene under the mec-3 promoter in the lite-1(xu7)mec-4(e1611) background. We analysed PVD-positive animals with FLP killed by laser. Control animals were transgene-free siblings. ** P <0.0001 ( t -test). n ≥5. Error bars: s.e.m. ( d ) ChR2 stimulation of PHA/PHB can drive forward movement. ChR2 was expressed as a transgene under the ocr-2 promoter in the lite-1(xu7) background [31] . To avoid turning on the head neurons labelled by the ocr-2 promoter, we directed light pulses to the animal tail. Control animals were transgene-free siblings. ** P <0.0001 ( t -test). n ≥5. Error bars: s.e.m. Full size image Similarly, ChR2 stimulation of the posterior sensory neurons PVD can trigger forward movement ( Fig. 4c ). A similar observation was made in animals expressing ChR2 in the anus sensory neuron PHA/PHB ( Fig. 4d ). However, we did not observe such a phenomenon in animals expressing ChR2 in PDE. It is possible that ChR2-mediated cation influx cannot fully mimic the kinetics and/or ion selectivity of the conductance carried by the endogenous mechanosensitive channels in these neurons. Nonetheless, these results provide additional evidence supporting a role for the identified sensory neurons in harsh touch sensation. A mechano-TRP channel regulates harsh touch sensation We next asked what genes are important for harsh touch sensation. The fact that animals lacking the gentle touch channel MEC-4/MEC-10 are sensitive to harsh touch suggests that other types of channels could be involved. TRP family channels are conserved between C. elegans and humans [25] . Many TRP channels have been implicated in mechanosensation, although the exact role of these channels in mechanosensation remains largely unclear [26] , [27] . The C. elegans genome encodes 17 TRP channel homologues covering all of the seven TRP subfamilies [28] , [29] . As the expression patterns of most TRP channels have been reported [28] , [29] , we examined those known to be expressed in harsh touch sensory neurons, including TRPV (OSM-9 and OCR-2), TRPA (TRPA-1) and TRPN (TRP-4) channels. TRPV channels have been implicated in mechanosensation in both invertebrates and vertebrates [27] , [30] . The C. elegans TRPV channel OCR-2 is expressed in the anus sensory neurons PHA/PHB and is required for mechanosensation mediated by the head neuron ASH [31] . We did not detect a defect in anus response in ocr-2 mutant animals ( Supplementary Fig. S8a ); nor did we observe a deficit in posterior response ( Supplementary Fig. S8b ). A similar result was obtained with animals lacking OSM-9, another TRPV channel expressed in PHA/PHB [32] , as well as animals lacking both OSM-9 and OCR-2 ( Supplementary Fig. S8 ). Thus, OCR-2/OSM-9 channels are not essential for anus harsh touch sensation. TRPA channels have been implicated in mechanosensation in both invertebrates and vertebrates [27] , [33] , [34] , [35] . The TRPA channel TRPA-1 is expressed in the anus sensory neurons PHA/PHB and posterior sensory neurons PVD and PDE [35] . However, we did not observe a noticeable defect in anus response; nor did we detect a phenotype in posterior response, suggesting that TRPA-1 may not be required for harsh touch sensation in these areas ( Fig. 5 and Supplementary Fig. S8 ). 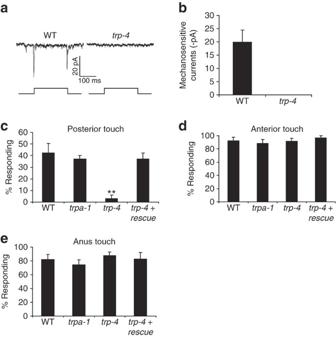Figure 5: The TRPN channel TRP-4 regulates posterior harsh touch response. (a) Touch evokes mechanosensitive currents in PDE in a TRP-4-dependent manner. Clamping voltage: −75 mV. Touch was directed to the cilium of PDE. Displacement: 10 μm. A displacement of 1 μm was sufficient to evoke mechanosensitive currents in PDE. (b) Bar graph summarizing the data in (a).n≥5. Error bars: s.e.m. (c) TRP-4 is required for posterior harsh touch behavioural response mediated by PDE. To rescue the defect, wild-typetrp-4cDNA was expressed as a transgene in PDE under thedat-1promoter intrp-4(sy695)mutant animals20,46. PVD and PLM were both killed in each genotype. **P<0.0001 (ANOVA with Bonferroni test compared with WT).n≥7. Error bars: s.e.m. (d) Responses to anterior harsh touch in worms described in (c). (e) Responses to anus harsh touch in worms described in (c). WT, wild type. Figure 5: The TRPN channel TRP-4 regulates posterior harsh touch response. ( a ) Touch evokes mechanosensitive currents in PDE in a TRP-4-dependent manner. Clamping voltage: −75 mV. Touch was directed to the cilium of PDE. Displacement: 10 μm. A displacement of 1 μm was sufficient to evoke mechanosensitive currents in PDE. ( b ) Bar graph summarizing the data in (a). n ≥5. Error bars: s.e.m. ( c ) TRP-4 is required for posterior harsh touch behavioural response mediated by PDE. To rescue the defect, wild-type trp-4 cDNA was expressed as a transgene in PDE under the dat-1 promoter in trp-4(sy695) mutant animals [20] , [46] . PVD and PLM were both killed in each genotype. ** P <0.0001 (ANOVA with Bonferroni test compared with WT). n ≥7. Error bars: s.e.m. ( d ) Responses to anterior harsh touch in worms described in ( c ). ( e ) Responses to anus harsh touch in worms described in ( c ). WT, wild type. Full size image TRPN channels have also been implicated in mechanosensation in a number of invertebrate and vertebrate organisms, including C. elegans , Drosophila and zebra fish [20] , [27] , [36] , [37] , [38] . The C. elegans TRPN channel TRP-4 represents the first-identified TRP family member that functions as a mechanically gated channel [39] . TRP-4 is required for proprioception mediated by the DVA neuron [20] . However, trp-4 mutant animals did not exhibit a defect in anus response ( Fig. 5e ). TRP-4 is also expressed in dopamine neurons, including PDE [20] , [36] . We therefore recorded PDE in response to touch by patch clamp. A glass probe driven by a piezo actuator was used to deliver touch to the cilium of PDE [39] . Similar to the other dopamine neuron CEP [39] , mechanical stimulation of the cilium of PDE evoked mechanosensitive currents with both an “on” and “off” response in a TRP-4-dependent manner ( Fig. 5a,b ). We further asked whether TRP-4 has a role in posterior harsh touch behaviour. To eliminate functional redundancy from PVD that does not seem to express TRP-4 ( Supplementary Fig. S8d ), we tested PVD-ablated animals and found that trp-4 mutant animals lost posterior response ( Fig. 5c ). As a control, no such defect was detected in trpa-1 mutant animals ( Fig. 5c ). Importantly, expression of wild-type trp-4 complementary DNA in PDE fully rescued the phenotype ( Fig. 5c ). We did not test the role of TRP-4 in ADE, as it is merely one of the five anterior sensory neurons; however, presumably, TRP-4 may have a similar role in this neuron. These observations indicate that TRP-4 regulates harsh touch sensation at least posteriorly. Amiloride-sensitive channels mediate mechano-currents in PVD We also recorded by patch clamp the mechanosensitivity of PVD, the other posterior sensory neuron. Mechanical stimulation of the dendrite of PVD evoked mechanosensitive currents with “on” and “off” components ( Fig. 6a ). Unlike dopamine neurons [39] , mechanosensitive currents in PVD are amiloride-sensitive ( Fig. 6b ). The amiloride sensitivity suggests that the channel is encoded by a member(s) in the ENaC family as reported for gentle-touch neurons [8] . Indeed, PVD mechanosensitive currents were inwardly rectifying with a reversal potential around +70 mV, close to the equilibrium potential of Na + , consistent with the view that they are carried by an ENaC channel(s) ( Fig. 6c ). 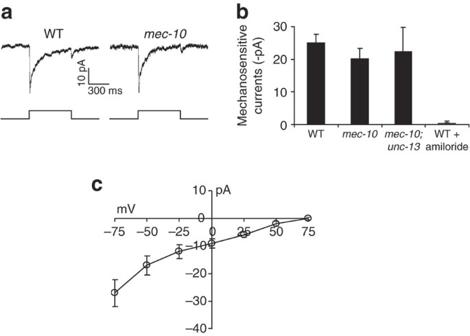Figure 6: An amiloride-sensitive channel(s) mediates mechanosensitive currents in PVD. (a) Mechanical stimulation evokes mechanosensitive currents in PVD. Such currents persisted inmec-10(tm1552). Clamping voltage: −75 mV. Touch was directed to the primary dendrite of PVD. Displacement: 20 μm. A 10-μm displacement was needed to evoke mechanosensitive currents in PVD, a much higher threshold than that in PDE. PVD inmec-10(tm1552)animals displayed a similar sensitivity (threshold). (b) Bar graphs. Touch-evoked mechanosensitive currents in PVD were sensitive to amiloride (200 μM) but persisted inmec-10(tm1552), as well as inmec-10(tm1552); unc-13(e51)double mutant animals.n≥5. Error bars: s.e.m. (c) I-V relations of mechanosensitive currents in PVD.n≥5. Error bars: s.e.m. Figure 6: An amiloride-sensitive channel(s) mediates mechanosensitive currents in PVD. ( a ) Mechanical stimulation evokes mechanosensitive currents in PVD. Such currents persisted in mec-10(tm1552) . Clamping voltage: −75 mV. Touch was directed to the primary dendrite of PVD. Displacement: 20 μm. A 10-μm displacement was needed to evoke mechanosensitive currents in PVD, a much higher threshold than that in PDE. PVD in mec-10(tm1552) animals displayed a similar sensitivity (threshold). ( b ) Bar graphs. Touch-evoked mechanosensitive currents in PVD were sensitive to amiloride (200 μM) but persisted in mec-10(tm1552) , as well as in mec-10(tm1552); unc-13(e51) double mutant animals. n ≥5. Error bars: s.e.m. ( c ) I-V relations of mechanosensitive currents in PVD. n ≥5. Error bars: s.e.m. Full size image The above result prompted us to examine MEC-10, an ENaC channel recently found to be essential for PVD mechanosensitivity in a calcium imaging assay [12] . Notably, mechanosensitive currents remained in the PVD of mec-10(tm1552) mutant animals ( Fig. 6a,b ). These mutant animals also retained behavioural responses to harsh touch ( Supplementary Fig. S9 ). The mechanosensitive currents in PVD persisted in mec-10;unc-13 double mutant animals in which synaptic transmission was abrogated, indicating that the recorded currents originated in PVD ( Fig. 6b ). We did not examine the other candidate mechanosensitive ENaC channel DEGT-1 expressed in PVD [12] , as no mutant is available for this channel. It is possible that another ENaC channel or DEGT-1 carries the mechanosensitive currents in PVD; alternatively, multiple ENaC channels may function redundantly in PVD. The discrepancy in MEC-10 between the two studies may result from the use of different functional and behavioural assays. Animals lacking harsh touch neurons respond to gentle touch Considering the fact that gentle touch-insensitive mutant animals are sensitive to harsh touch, one might ask whether animals lacking harsh touch sensory neurons respond to gentle touch. To test this, we ablated all of the anterior harsh touch sensory neurons, but left intact the anterior gentle touch sensory neurons ALM and AVM. These animals responded normally to anterior gentle touch ( Fig. 7a ). We also killed the posterior harsh touch sensory neurons PVD and PDE, but spared the posterior gentle touch neuron PLM. These animals responded normally to posterior gentle touch ( Fig. 7b ). Thus, animals lacking harsh touch sensory neurons retained gentle touch responses, providing additional evidence that C. elegans uses distinct sensory neurons to detect harsh touch and gentle touch. 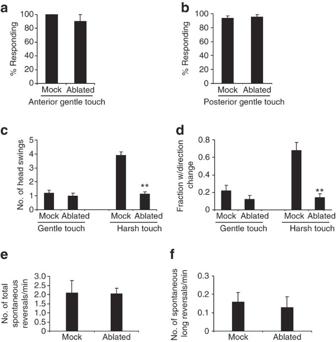Figure 7: Animals lacking harsh touch sensory neurons can no longer distinguish harsh touch from gentle touch. (a) Worms lacking anterior harsh touch sensory neurons retain sensitivity to anterior gentle touch. All five anterior sensory neurons (BDU, SDQR, FLP, ADE and AQR) were ablated. Anterior gentle touch neurons (ALM and AVM) were not killed.n=10. Error bars: s.e.m. (b) Worms lacking posterior harsh touch sensory neurons retain sensitivity to posterior gentle touch. PDE and PVD were ablated. The posterior gentle touch neuron PLM was not killed.n=10. Error bars: s.e.m. (c) Worms lacking harsh touch sensory neurons responded similarly to harsh touch and gentle touch. All anterior harsh touch sensory neurons were ablated, and the ablated animals were assayed for anterior gentle and harsh touch responses. The number of head swings of backward movement triggered by anterior harsh and gentle touch was scored. Gentle touch sensory neurons were not killed.n=10. **P<0.0001 (ANOVA with Bonferroni test compared with mock). Error bars: s.e.m. (d) The same worms in (c) were scored for the frequency of direction change following backward movement.n=10. **P<0.0001 (ANOVA with Bonferroni test compared with mock). Error bars: s.e.m. (e) Animals lacking all anterior harsh touch sensory neurons show a normal frequency of spontaneous reversals.n=10. Error bars: s.e.m. (f) Animals lacking all anterior harsh touch sensory neurons show a normal frequency of long reversals during spontaneous locomotion. Long reversals are defined as backward movement events with >3 head swings.n=10. Error bars: s.e.m. Figure 7: Animals lacking harsh touch sensory neurons can no longer distinguish harsh touch from gentle touch. ( a ) Worms lacking anterior harsh touch sensory neurons retain sensitivity to anterior gentle touch. All five anterior sensory neurons (BDU, SDQR, FLP, ADE and AQR) were ablated. Anterior gentle touch neurons (ALM and AVM) were not killed. n =10. Error bars: s.e.m. ( b ) Worms lacking posterior harsh touch sensory neurons retain sensitivity to posterior gentle touch. PDE and PVD were ablated. The posterior gentle touch neuron PLM was not killed. n =10. Error bars: s.e.m. ( c ) Worms lacking harsh touch sensory neurons responded similarly to harsh touch and gentle touch. All anterior harsh touch sensory neurons were ablated, and the ablated animals were assayed for anterior gentle and harsh touch responses. The number of head swings of backward movement triggered by anterior harsh and gentle touch was scored. Gentle touch sensory neurons were not killed. n =10. ** P <0.0001 (ANOVA with Bonferroni test compared with mock). Error bars: s.e.m. ( d ) The same worms in ( c ) were scored for the frequency of direction change following backward movement. n =10. ** P <0.0001 (ANOVA with Bonferroni test compared with mock). Error bars: s.e.m. ( e ) Animals lacking all anterior harsh touch sensory neurons show a normal frequency of spontaneous reversals. n =10. Error bars: s.e.m. ( f ) Animals lacking all anterior harsh touch sensory neurons show a normal frequency of long reversals during spontaneous locomotion. Long reversals are defined as backward movement events with >3 head swings. n =10. Error bars: s.e.m. Full size image But these animals interpret harsh touch as gentle touch Having demonstrated that animals lacking harsh touch sensory neurons retained gentle touch responses, we wondered how these animals respond to harsh touch ( Fig. 7c–f ). Again, we focused on the anterior response by quantifying the number of head swings of backward movement triggered by anterior harsh and gentle touch. In ablated animals (lacking anterior harsh touch neurons but retaining anterior gentle touch neurons), the number of head swings evoked by harsh touch was similar to that triggered by gentle touch ( Fig. 7c ). This defect was not caused by an inability of ablated animals in executing long reversals, as they exhibited long reversals in spontaneous locomotion at a frequency similar to that observed in mock-ablated animals ( Fig. 7f ). In addition, following reversals, ablated animals typically moved forward without a change in direction, a phenomenon resembling gentle touch response ( Fig. 7d ). These results suggest that animals lacking harsh touch sensory neurons can no longer distinguish harsh touch from gentle touch, providing further evidence that C. elegans uses distinct sensory neurons to sense harsh touch and gentle touch. A neuronal correlate for harsh and gentle touch sensation Finally, we explored the neural basis by which C. elegans distinguishes harsh touch from gentle touch. Clearly, the interneurons mediating gentle and harsh behaviour largely overlap. This suggests that gentle and harsh touch sensory neurons may send differential outputs to the interneurons. We tested this model on the interneuron PVC, as we found it relatively easy to record the response of this neuron to touch by calcium imaging. Both gentle and harsh touch can stimulate PVC ( Fig. 8a,b ). Importantly, the amplitude of PVC calcium response evoked by harsh touch was significantly greater than that induced by gentle touch ( Fig. 8a,b ). This is consistent with our behavioural data showing that harsh touch responses were more robust than gentle touch responses. 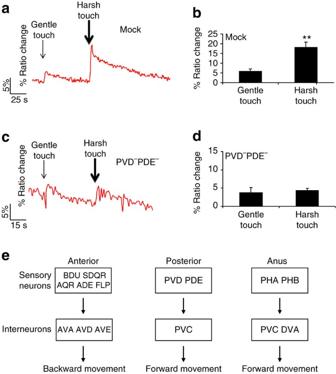Figure 8: Differential stimulation of the interneuron PVC by gentle and harsh touch. (a) Harsh touch evokes a greater calcium response in PVC. Gentle touch (5 μm at 20 Hz; 3 s) and harsh touch (20 μm at 20 Hz; 3 s) were sequentially delivered to the posterior body of immobilized animals. (b) Bar graph summarizing the data in (a). **P<0.0001 (t-test).n=21. Error bars: s.e.m. (c) Animals lacking harsh touch sensory neurons responded similarly to harsh and gentle touch in PVC. (d) Bar graph summarizing the data in (c).n=5. Error bars: s.e.m. (e) A diagram summarizing the neural circuits underlying harsh touch sensation. The sensory neurons and interneurons required for harsh touch sensation in each body segment are listed. Figure 8: Differential stimulation of the interneuron PVC by gentle and harsh touch. ( a ) Harsh touch evokes a greater calcium response in PVC. Gentle touch (5 μm at 20 Hz; 3 s) and harsh touch (20 μm at 20 Hz; 3 s) were sequentially delivered to the posterior body of immobilized animals. ( b ) Bar graph summarizing the data in ( a ). ** P <0.0001 ( t -test). n =21. Error bars: s.e.m. ( c ) Animals lacking harsh touch sensory neurons responded similarly to harsh and gentle touch in PVC. ( d ) Bar graph summarizing the data in ( c ). n =5. Error bars: s.e.m. ( e ) A diagram summarizing the neural circuits underlying harsh touch sensation. The sensory neurons and interneurons required for harsh touch sensation in each body segment are listed. Full size image As our behavioural experiments revealed that animals lacking harsh touch sensory neurons interpret harsh touch as gentle touch, we sought to provide a neuronal correlate for this observation. We repeated the calcium imaging experiment on animals lacking the posterior harsh touch sensory neurons ( Fig. 8c,d ). PVC in these animals no longer displayed differential calcium responses to gentle and harsh touch but instead responded similarly to these two types of stimuli ( Fig. 8c,d ), providing a neuronal correlate for our behavioural observation. In this study, we show that C. elegans exhibits differential behavioural responses to harsh touch and gentle touch, an observation also seen in higher organisms [2] . The fact that C. elegans exhibits robust harsh touch responses may allow it to effectively avoid this hazardous cue, providing a mechanism for its survival. C. elegans recruits a distinct set of sensory neurons to detect harsh touch, a phenomenon that is also observed in higher organisms ( Fig. 8e ). Thus, harsh touch sensation in nematodes and mammals appears to bear some interesting analogies at the behavioural and neural circuit level. Unlike gentle touch sensory neurons that all belong to the same class of non-ciliated neurons containing 15-protofilament microtubules [1] , the sensory neurons required for harsh touch sensation include both ciliated and non-ciliated cells. Despite this morphological difference, many of these neurons share the same precursors in lineage, and some are in fact sister neurons. For example, the posterior sensory neuron PVD and PDE are both descendents of V5; BDU and ALM are sister neurons; and SDQR and AVM share the same precursor QL [19] . It is not clear whether this contributes to their functional identity in touch sensation. PVD and FLP are both multidendritic neurons [17] , with one involved in detecting posterior touch and the other in anterior touch. As the dendrites of these neurons cover a large surface area of C. elegans body, they may possess a large receptive field. Then how would ciliated neurons compensate for the small size of their sensory cilia? Notably, the sensory cilia of ciliated neurons such as PDE exhibit a higher mechanosensitivity than the dendrites of PVD. Unlike that in patch-clamp recordings, in behavioural assays the majority of touch stimuli are probably delivered at a position quite distant to rather than right on top of the cilia; in this case, their high mechanosensitivity would allow them to sense those nearby or distantly positioned touch stimuli. In this regard, these ciliated neurons may also be considered as light-touch neurons that sense harsh touch in distance. Finally, it should be noted that although we have identified the sensory neurons required for harsh touch sensation, whether they all are truly mechanosensory neurons such as PVD and PDE require functional confirmation, and we also do not exclude the possibility that other sensory neurons may have a role in this behaviour. Unlike sensory neurons, the interneurons required for harsh touch and gentle touch behaviours largely overlap, suggesting that these interneurons may receive differential inputs from gentle and harsh touch sensory neurons. This model is supported by calcium imaging analysis of the interneuron PVC in response to gentle and harsh touch. This suggests that the sensory information may be encoded at least partly in the sensory neurons in the posterior circuit. The observation that gentle touch mutants are sensitive to harsh touch suggests that C. elegans may not rely on the same genes to regulate harsh touch responses. Indeed, we show that both TRP and ENaC family channels are involved in regulating harsh touch sensation. Although the activity of mechanically-gated channels has been detected in many cell types in metazoans, very little is known about their molecular identities [27] , [30] . The ENaC family channel MEC-4/MEC-10, K2P channel TREK-1, newly identified Piezos, and TRPN (TRP-NOMPC) family channel TRP-4 arguably represent the only exceptions [30] , [39] , [40] . We have tested a number of TRP channel mutants in harsh touch behaviour. Although most of the tested TRP channels are not essential for behavioural responses to harsh touch, it does not preclude the possibility that they do have a role in harsh touch sensation. The identification of TRP and ENaC family channels provides a proof-of-principle that C. elegans can be used as a model to identify genes regulating harsh touch sensation. Our studies lay the foundation for future work that promises to elucidate the molecular mechanisms underlying harsh touch sensation in C. elegans , which may facilitate our understanding of this sensory modality in higher organisms. Strains Wild type: N2 . CB1338: mec-3(e1338) —CGC strain, not outcrossed. TQ526: mec-3(e1338) ×4 outcrossed. TQ1243: mec-4(e1611) ×6 outcrossed. TQ428: akIs3[Pnmr-1 ∷ gfp] ×8 outcrossed. TQ509: daf-19(m86); mec-4(e1611). TQ519: xuEx320[Pmec-3 ∷ gfp; Pdat-1 ∷ yfp2; Pdat-1 ∷ dsred]. TQ945: xuEx16[Pgcy-35 ∷ yfp+Pmec-3 ∷ gfp]. TQ1380: xuEx847[Ptwk-16 ∷ dsred]. TQ1415: xuEx471[Pdat-1 ∷ dsred+Punc-122 ∷ gfp]. TQ1991: xuEx536[Pmec-3 ∷ dsred+Pocr-2 ∷ dsred]; xuEx320. TQ1436: xuEx368[Pdat-1 ∷ ChR2+Pdat-1 ∷ dsred+lin-15(+)]; lite-1(xu7). TQ1438: xuEx474[Pocr-2 ∷ ChR2+Pocr-2 ∷ dsred+lin-15(+)]; lite-1(xu7). TQ1443: xuEx479[Pgcy-35 ∷ ChR2+Pgcy-35 ∷ dsred+lin-15(+)]; lite-1(xu7). TQ1576: lite-1(xu7); mec-4(e1611); xuEx531[Pmec-3 ∷ ChR2+Pmec-3 ∷ dsred+lin-15(+)]. TQ1737: trp-4(sy695); xuEx584[Pdat-1 ∷ trp-4 ∷ SL2 ∷ yfp+Punc-122 ∷ gfp]; xuEx12. TQ1732: trp-4(sy695); xuEx320. TQ1569: mec-10(tm1552); xuEx320. TQ1988: trpa-1(ok999); xuEx320. TQ1989: ocr-2(ak47); xuEx320. TQ1990: osm-9(ky10); xuEx320. TQ2177: ocr-2(ak47)osm-9(ky10); xuEx320. TQ2179: mec-10(tm1552); unc-13(e51); xuEx12. TQ2290: lite-1(xu7); xuEx648[Pnmr-1 ∷ G-CaMP3.0+Pnmr-1 ∷ dsred]; xuEx471 . Behavioural analysis and molecular biology Harsh touch was delivered with a platinum wire pick (2 cm in length, 99.95% purity, 0.25 mm in diameter; cat# PTP101 from WPI) mounted to a glass Pasteur pipette. The tip of the pick was flattened to 20 μm in thickness and cut to make an edge with a width of 30 μm. We touched the worm body with the edge in a top-down manner. One should avoid scratching the surface of the assay plate. One hour before testing, day-1 adult animals were transferred to an Nematode Growth Medium (NGM) plate spread with a thin layer of freshly grown OP50 bacteria. Each worm was tested five times with a 2–10 min interval between each trial, and a response rate for each worm was tabulated. We tested anterior response on animals slowly moving forward, and examined posterior, anus and middle-segment (vulva touch) responses on animals that were non-moving or nearly non-moving. To estimate forces, we touched animals on an NGM testing plate, which was placed on top of an analytical balance. The applied forces can be estimated by recording the readings on the analytical balance. In this case, the worm was semi-immobilized by gluing its vulva area with cyanoacrylate glue to facilitate force recording. This protocol estimated that the average force applied to the anterior, posterior and anus area was: 140±40 μN, 150±30 μN, and 80±40 μN, respectively ( n =10 each, ± indicates s.d.). Before scoring freely moving animals, we found it helpful to practise touching animals on an analytical balance. We recommend not starting to score animals unless the practice shows that applied forces are within the range as listed above. Gentle touch was delivered with an eyelash. mec-4 mutant animals may respond to some “stiff” eyelash if large forces are applied. Thus, before each new experiment, we always practiced on both wild-type and mec-4 mutant animals to ensure that wild-type animals responded but mec-4 animals did not. To quantify spontaneous reversal rate, we used an automated worm tracking system [41] , [42] . Day-1 adult animals were tracked for 10 min on NGM plates spread with a thin layer of freshly-grown OP50 bacteria. Laser ablation was performed on L1-L3 animals with a MicroPoint Laser system (Photonic Instruments) on 2% agarose pad, and ablated animals were allowed to grow to adulthood before behavioural analysis [43] ( Supplementary Fig. S10 ). A green fluorescent protein transgene driven by the nmr-1 promoter was used to aid ablation of interneurons [44] . To ablate BDU, SDQ, AQR and PQR, we used a YFP transgene driven by the gcy-35 promoter [45] . A green fluorescent protein transgene under the mec-3 promoter was used to ablate gentle touch neurons and PVD and FLP [11] , and a similar transgene under the dat-1 promoter was used to help ablate PDE and ADE [46] . To ablate PHA/PHB, we used a green fluorescent protein transgene expressed under the ocr-2 promoter [31] . To rescue the trp-4 phenotype in PDE, wild-type trp-4 cDNA was expressed as a transgene under the dat-1 promoter [46] , and the plasmid was directly injected into the trp-4(sy695) mutant background. Optogenetics Animals were grown on NGM plates containing 5 μM of all-trans retinal. Day-1 adult animals were tested on retinal-free plates spread with a thin layer of freshly grown OP50 bacteria. All experiments were performed on lite-1(xu7) animals that lack intrinsic phototaxis responses to short-wavelength light [4] , [5] . Each worm was tested five times with a 5–8 min interval between each trial, and a response rate was tabulated for each worm. Blue light pulses (2 s from an EXFO Xcite lamp) at an intensity of 5–10 mW mm −2 were delivered to the anterior, posterior or tail of the worm via an ×10 objective in combination with a zoom lens on a Zeiss microscope (Zeiss Discovery). We closed the diaphragm of the microscope to direct light to individual body parts. To test posterior and anus responses, we challenged non-moving animals. A positive response was scored if the animal began to move forward (for posterior and anus responses) or stopped forward movement (for anterior response) within 3 s after the cessation of light illumination and also initiated backward movement that lasted at least half a head swing. Background light used to visualize animals was filtered into red. Light intensity was determined with a radiometric sensor head (268LP) coupled to an optometer (S471; UDT Instruments). Electrophysiology and calcium imaging Whole-cell recordings were performed on an Olympus microscope (BX51WI) with an EPC-10 amplifier controlled by the Patchmaster software (HEKA). A glass stimulus probe was driven by a Piezo actuator (PI) mounted on a micromanipulator (Sutter). Animals were glued to a sylgard-coated coverglass covered with bath solution, and a small piece of cuticle in the posterior body was cut open and pinned down to the coverglass to expose the cell body of PDE and PVD, which can be identified by a green or red fluorescent protein marker expressed as a transgene driven by the dat-1 and mec-3 promoter, respectively [11] , [47] . Touch was directed to the cilium of PDE or primary dendrite of PVD by pressing the cuticle overlaying the cilium or primary dendrite, respectively. Recording pipettes were pulled from borosilicate glass. The bath solution contains 145 mM NaCl, 10 mM HEPES, 20 mM glucose, 1 mM MgCl 2 , 1 mM CaCl 2 , and 2.5 mM KCl (335 mOsm; pH adjusted to 7.3 with NaOH). The pipette solution contains 145 mM CsCl, 10 mM HEPES, 20 mM glucose, 0.25 mM CaCl 2 , and 5 mM EGTA, 5 mM Na 2 ATP, 0.5 mM GTP (325 mOsm; pH adjusted to 7.2 with CsOH). Voltages were clamped at -75 mV. Current data were sampled at 20–40 kHz. Series resistance and membrane capacitance were both compensated during recording. Liquid junction potentials were also corrected. Calcium imaging was performed on the same hardware system used for patch-clamp recording. MetaFlour (Molecular Devices) was used for imaging acquisition and analysis. G-CaMP3.0 and DsRed2 were co-expressed in PVC as a transgene driven by the nmr-1 promoter to allow for ratiometric imaging. Animals were immobilized on a 5% agarose pad with cyanoacrylate glue in bath solution containing 2.5 mM serotonin. G-CaMP and DsRed2 fluorescence was excited at 484 nm and 565 nm, respectively. The peak percentage ratio change (484/565 nm) was used to quantify calcium levels in PVC. How to cite this article: Li, W., et al . The neural circuits and sensory channels mediating harsh touch sensation in C. elegans . Nat. Commun. 2:315 doi: 10.1038/ncomms1308 (2011).